Fringing-field dielectrophoretic assembly of ultrahigh-density semiconducting nanotube arrays with a self-limited pitch One key challenge of realizing practical high-performance electronic devices based on single-walled carbon nanotubes is to produce electronically pure nanotube arrays with both a minuscule and uniform inter-tube pitch for sufficient device-packing density and homogeneity. Here we develop a method in which the alternating voltage-fringing electric field formed between surface microelectrodes and the substrate is utilized to assemble semiconducting nanotubes into well-aligned, ultrahigh-density and submonolayered arrays, with a consistent pitch as small as 21±6 nm determined by a self-limiting mechanism, based on the unique field focusing and screening effects of the fringing field. Field-effect transistors based on such nanotube arrays exhibit record high device transconductance (>50 μS μm −1 ) and decent on current per nanotube (~1 μA per tube) together with high on/off ratios at a drain bias of −1 V. Semiconducting single-walled carbon nanotubes are poised to replace silicon in high-performance microprocessor chips and are expected to offer a significant improvement in energy-delay product [1] , [2] , [3] , [4] , based on their attractive electrical properties demonstrated in field-effect transistors (FETs) constructed on individual nanotubes, especially their good electrical contacts with metals and their atomically smooth intrinsic ultrathin body [5] , [6] , [7] . However, in a technological application, transistors must rely on an array of parallel nanotubes to deliver sufficient current output. Therefore, the distance between neighbouring nanotubes has to be small enough to enable the high device-packing density. In addition, the inter-tube pitch also needs to be consistent for achieving the level of device uniformity and yield required for ultra-large-scale circuit integration [8] . Although significant progress has been made in aligning nanotubes, a method that can produce submonolayered semiconducting nanotube arrays with both a tight and uniform pitch has not yet been demonstrated. Guided by anisotropic interaction between nanotubes and certain single-crystalline substrates, sparse arrays of long nanotubes can be grown by chemical vapour deposition (CVD), with their pitch widely distributed in the 100–500-nm range after the selective removal of metallic nanotubes during or after synthesis [9] , [10] , [11] . Rather than using the selective etching schemes, nanotubes can also be first sorted in solution and then assembled into regular arrays. Although these chemically purified solution tubes demonstrate lower intrinsic mobility than that of CVD tubes, they have identical ultrathin body and similar contact resistance with electrodes, which has been experimentally shown to be about an order of magnitude larger than the channel resistance if the device gate length is scaled to ~10 nm [12] . Therefore, ultrascaled transistors based on such solution nanotubes yield performance and variability comparable to that obtained with CVD tubes, as the device operation is largely limited by the short channel effects and the contacts rather than the channel in this regime [6] . In one example, semiconducting nanotube arrays can be generated by utilizing chemical recognition between pre-sorted nanotubes and pre-patterned functionalized substrates [13] , [14] , [15] . This method provides a tighter pitch control, but the smallest pitch that has ever been reported is >200 nm. Further reduction of pitch and narrowing its distribution with this approach could be challenging, owing to the undefined inter-tube interactions within a trench and the defects from nanotubes bridging across trenches. The Langmuir–Schaefer method has recently been exploited to form densely aligned nanotube arrays in which nanotubes are arranged in an unoptimized double-layered structure, which could be detrimental to device operations due to electrostatic screening [16] . Deoxyribonucleic acid linkers or depletion attraction forces during solvent evaporation assemble nanotubes into rafts of aligned arrays [17] , [18] . However, the fact that their alignment directions and locations on the substrate cannot be precisely controlled makes these methods less attractive for practical applications. Alternating voltage dielectrophoresis is a very versatile methodology to pattern nanomaterials, including nanoparticles, nanowires and biomacromolecules [19] , [20] , [21] . It utilizes an inhomogeneous electric field, typically formed between a pair of planar microelectrodes, to manipulate the placement of nanomaterials via interaction with their induced dipole moment [22] . However, limited success has been achieved with carbon nanotubes. Assembled arrays are typically rich of various curving and wiggling defects due to random hydrodynamic force and Brownian motion of nanotubes. More importantly, the formation of commonly observed multilayer defects makes it almost impossible to achieve a meaningful inter-tube pitch of <40 nm or any pitch uniformity control [23] , [24] , [25] , [26] . Here we investigate the use of the fringing electric field formed between surface microelectrodes and the substrate to assemble carbon nanotubes by dielectrophoresis. The strong field-focusing effect of the fringing field leads to very high alignment force and ensures the formation of nearly perfectly aligned arrays of highly linear nanotubes. At the same time, a self-limiting mechanism based on the effective screening of the fringing electric field by deposited nanotubes guarantees the formation of submonolayered structure with a precisely defined uniform pitch over a wide process window. This process is compatible with established semiconducting nanotube-sorting techniques [27] , [28] , [29] , and has the scalability to cover the majority of a wafer surface with assembled nanotube arrays (see Supplementary Fig. 1 ; Supplementary Note 1 ). Fringing-field dielectrophoretic assembly of nanotubes The setup and process of the fringing-field dielectrophoretic nanotube assembly are conceptually illustrated in Fig. 1a . The important feature of this setup compared with conventional planar dielectrophoresis is that all the microelectrodes patterned on top of a thin 10-nm-thick thermal silicon oxide are wired together, while the underlying grounded silicon substrate serves as the counter electrode. Metal electrodes are further protected with a thin, c.a.~8 nm, layer of Al 2 O 3 deposited by atomic layer deposition to avoid potential material issues such as electromigration associated with heat dissipation during dielectrophoresis [25] . A few drops of dialysed SDS-nanotube suspension are applied onto the chip as the nanotube reservoir. Dialysis removes extra ionic surfactant from the nanotube suspension, providing lower ionic concentration, which minimizes ionic relaxation. It allows for dielectrophoretic assembly at a low-enough frequency, where the dielectrophoretic force is independent of nanotube permittivity so that both metallic and semiconducting nanotubes can be deposited simultaneously [30] . It also reduces the solution conductivity ( σ sol ) and therefore increases the magnitude of the dielectrophoretic force on the nanotubes, which is proportional to ( σ tube − σ sol )/ σ sol , where σ tube is the conductivity of carbon nanotubes [22] . A function generator supplies the alternating voltage signal (sinusoid with a peak-to-peak voltage of 5 V and a frequency of 400 kHz) to the electrodes for 4 min, and a final wash with deionized water completes the assembly process. The fringing field formed between the microelectrode arrays and the silicon substrate exerts a time-averaged dielectrophoretic force on the nanotubes, forcing them to align with electric lines of force, which are perpendicular to the edge of the microelectrodes, and move downwards to the surface along the gradient as shown in Fig. 1b,c . The alignment direction of the nanotubes on the same substrate can be simply adjusted by modifying the shape of the assembly microelectrode. Possessing such a capability is also a significant advantage over some other assembly techniques, such as substrate-guided CVD growth and Langmuir–Schaefer assembly, as it allows greater freedom in circuit layout design. Assembled nanotube arrays have the option to be transferred to other substrates for subsequent device fabrications by wafer-scale transfer printing techniques [31] . 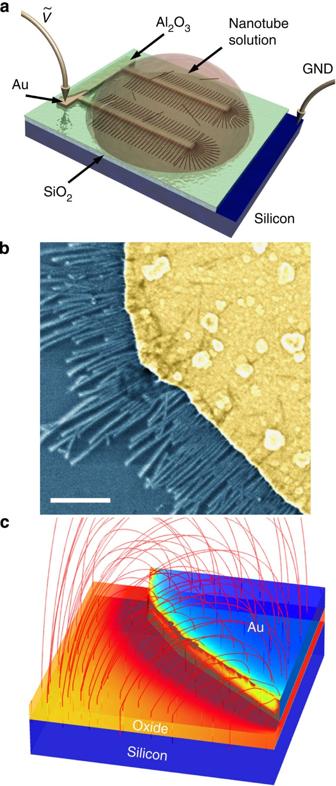Figure 1: Assembly of ultrahigh-density semiconducting nanotube arrays with the fringing-field dielectrophoresis. (a) Schematic illustration of the fringing-field dielectrophoretic nanotube assembly process. [Vtilde]: alternating voltage input. GND: electric ground. (b) False-coloured SEM image shows the assembled nanotube arrays with alignment direction controlled by the electric field distribution. Scale bar, 500 nm. (c) Three-dimensional finite-element method simulation depicts the fringing electric field formed between an assembly electrode and the Si substrate. Red colour intensity quantifies the strength of the electric field on the surface and red lines illustrate the electric field vectors in space. Figure 1: Assembly of ultrahigh-density semiconducting nanotube arrays with the fringing-field dielectrophoresis. ( a ) Schematic illustration of the fringing-field dielectrophoretic nanotube assembly process. [Vtilde]: alternating voltage input. GND: electric ground. ( b ) False-coloured SEM image shows the assembled nanotube arrays with alignment direction controlled by the electric field distribution. Scale bar, 500 nm. ( c ) Three-dimensional finite-element method simulation depicts the fringing electric field formed between an assembly electrode and the Si substrate. Red colour intensity quantifies the strength of the electric field on the surface and red lines illustrate the electric field vectors in space. Full size image Alignment and linearity of assembled nanotubes The quality of the assembled arrays is initially assessed through evaluating the alignment and linearity of the nanotubes. The fringing-field dielectrophoretic nanotube assembly yields a much higher degree of alignment, with virtually all nanotubes confined within ±6° of one another as shown in Fig. 2a , than those generated by other techniques for solution-processed nanotubes, including the planar dielectrophoresis, Langmuir–Schaefer method and chemical placement, where nanotubes are reported to lie within ±15°~±30° deviating from the major alignment direction [14] , [16] , [24] . Such high degree of alignment is also supported by the large, c.a. ~15, optical anisotropy observed in polarized Raman spectra (see Supplementary Fig. 2 ; Supplementary Note 2 ). In addition to misalignment, nanotube arrays assembled from their liquid suspensions generally suffer from significant curving and wiggling defects. However, nanotubes assembled by the fringing-field dielectrophoresis demonstrate nearly perfect linearity, with the deviation from a straight linear shape <20 nm. Both attributes result at least partially from the unique electric field-focusing effect of the fringing field formed between the assembly electrodes and the substrate separated by a very thin layer of dielectric [32] . Such a field-focusing effect leads to several times higher dielectrophoretic force and electro-orientation torque to place and align nanotubes compared with those of the planar dielectrophoresis according to finite-element simulations (see Supplementary Fig. 3 ; Supplementary Note 3 ). This large alignment force overwhelms disturbances from hydrodynamic force, Brownian motion and local heating of surrounding nanotube solution by microwave energy [33] , [34] , improving both alignment and linearity. In addition, the naturally formed dielectrophoretic force gradient extending from the edge of the microelectrodes could also contribute to the improvement of alignment and linearity of assembled nanotubes. While anchoring one end of the nanotube on the microelectrode, it allows the other end of the nanotube sufficient time to relax into its minimum energy position along the electric lines of force before the whole nanotube gets trapped on the surface by the van der Waals interaction. 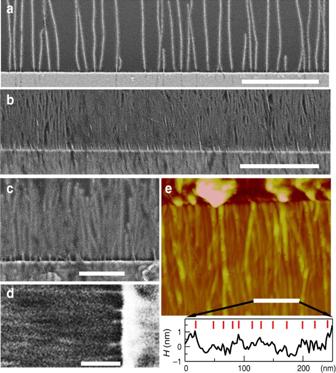Figure 2: Microscopic characterizations of the nanotube arrays assembled using the fringing-field dielectrophoresis. (a) SEM image of arrays assembled from dilute nanotube solution. Scale bar, 1 μm. (b–d) SEM images of arrays assembled from the concentrated nanotube solution with low (b, scale bar, 1 μm), medium (c, scale bar, 200 nm) and high (d, scale bar, 100 nm) magnifications. The height of the framedis 100 nm. (e) AFM image of ultrahigh-density semiconducting nanotube arrays. Scale bar, 250 nm. Bottom frame shows the magnified cross-sectional height (H) profile, with red lines as a visual guide marking the position of each nanotube inside the array. Figure 2: Microscopic characterizations of the nanotube arrays assembled using the fringing-field dielectrophoresis. ( a ) SEM image of arrays assembled from dilute nanotube solution. Scale bar, 1 μm. ( b – d ) SEM images of arrays assembled from the concentrated nanotube solution with low ( b , scale bar, 1 μm), medium ( c , scale bar, 200 nm) and high ( d , scale bar, 100 nm) magnifications. The height of the frame d is 100 nm. ( e ) AFM image of ultrahigh-density semiconducting nanotube arrays. Scale bar, 250 nm. Bottom frame shows the magnified cross-sectional height ( H ) profile, with red lines as a visual guide marking the position of each nanotube inside the array. Full size image Inter-tube pitch control The inter-nanotube pitch is another critical topological parameter for carbon nanotube arrays. Smaller pitch generally transfers to higher device performance. However, at the same time extra care must be taken to avoid the formation of multilayer defects, which could harm the device operation due to the screening of the gate electric field and the formation of transport barriers at tube–tube junctions [35] . In our fringing-field dielectrophoretic assembly setup, since all microelectrodes are biased at the same voltage, the deposition of one layer of nanotubes effectively screens the fringing field and makes the whole top surface of nearly equal potential. Therefore, the deposition of nanotubes is self-limited within a submonolayer (see Supplementary Figs 4 and 5 ; Supplementary Notes 4 and 5 ). This self-limiting mechanism allows us to push the nanotube density higher without worrying about the formation of multilayer defects. Figure 2b–d shows scanning electron microscopy (SEM) images of an ultra-dense 99% semiconducting nanotube array assembled from a semiconducting nanotube-enriched solution, prepared by column chromatography [28] , with a high concentration of 0.9 μg ml −1 (see Supplementary Fig. 6 ; Supplementary Note 6 ). The nanotube density is quite uniform over a large area as shown in the picture with a low magnification ( Fig. 2b ). The quality of nanotube alignment or linearity is not affected by the reduction of pitch distance, as shown in further zoomed-in images ( Fig. 2c,d ). A uniform pitch down to ~20 nm is revealed by both the magnified SEM ( Fig. 2d ) and the atomic force microscopy (AFM) images ( Fig. 2e ), representing the smallest pitch that has ever been demonstrated for large-area submonolayered semiconducting nanotube arrays. The height of most nanotubes ranges from 0.6 to 2 nm as measured by AFM, confirming the formation of the submonolayered structure. Some larger diameter nanotubes are likely from residual bundles present in the initial solution. In addition to reducing the smallest achievable pitch, the fringing-field dielectrophoretic assembly also improves the pitch consistency. In circuits, the pitch uniformity along with the pitch value determines the limit of the device footprint, as a high level of device uniformity is needed for integration. Quantitative analysis of the pitch uniformity of ultrahigh-density nanotube arrays assembled by the fringing-field dielectrophoresis is obtained from measuring the pitch among ~80 nanotubes, as shown in Fig. 3a ; Supplementary Fig. 7 , following the procedure described in Supplementary Note 7 . Most nanotubes are separated from their neighbours by 15~25 nm, with a s.d. as small as 6 nm, as depicted in Fig. 3b . This high degree of pitch uniformity, together with a small average pitch of 21 nm, makes it possible for nanotube FETs to achieve the channel resistance variability comparable to that of the 22-nm silicon finFET with identical device width. It marks an important step for the introduction of nanotubes into practical technological applications in terms of their variability performance, while additional efforts are still required to control the fluctuations of the threshold voltage and the contact resistance of nanotube transistors (see Supplementary Fig. 8 ; Supplementary Note 8 ). This tight pitch distribution is obtained based on the similar self-limiting mechanism but in three dimensions. As illustrated in Fig. 3c , the deposition of one nanotube effectively shields the electric field around it, and prevents the deposition of additional nanotubes too close to itself. We simulate the electric field distribution for different pitch values while keeping other geometrical parameters and the applied voltage identical to the values used in our experiments. The averaged force at the half-pitch position between two neighbouring nanotubes is plotted as a function of inter-tube pitch as shown in Fig. 3d . At large pitch, the fringing-field distribution and therefore the dielectrophoretic force near the central area is not affected. Additional nanotubes can still be deposited to reduce the pitch, up to the point where the dielectrophoretic force at the middle position of two neighbouring nanotubes starts to decay exponentially due to the screening of neighbouring nanotubes. This self-limiting mechanism prevents the deposition of another nanotube in between and locks the pitch to a fixed value. The fitted exponential time constant for this transition is at around 24±2 nm in this geometry according to the simulation, which agrees both qualitatively and quantitatively well with what we observed in experiments. Although further reduction of pitch is possible by modifying local electrostatics, the adoption of new chemistry for nanotube functionalizations is necessary to prevent the bundle formation at smaller pitch due to inter-tube π–π attractive interactions. 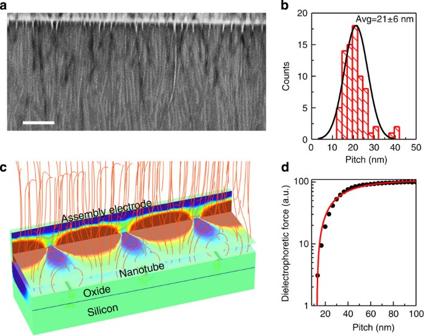Figure 3: Pitch uniformity of nanotube arrays assembled using the fringing-field dielectrophoresis. (a) Large area SEM image showing the uniformity of the nanotube pitch. Scale bar, 200 nm. (b) Statistical distribution of the pitch measured for ~80 nanotubes. Black solid line represents a Gaussian fitting. (c) Simulated three-dimensional distribution of dielectrophoretic force vectors for a given nanotube array with a uniform pitch of 66 nm. Red area indicates the existence of strong attractive dielectrophoretic force while the blue area is related with repulsive force. (d) The calculated average dielectrophoretic force at the half-pitch position between neighbouring nanotubes as a function of pitch values. Red line plots the fitting to a logarithmic decay function ofy=Ae−x/t, wheretis the exponential time constant. Figure 3: Pitch uniformity of nanotube arrays assembled using the fringing-field dielectrophoresis. ( a ) Large area SEM image showing the uniformity of the nanotube pitch. Scale bar, 200 nm. ( b ) Statistical distribution of the pitch measured for ~80 nanotubes. Black solid line represents a Gaussian fitting. ( c ) Simulated three-dimensional distribution of dielectrophoretic force vectors for a given nanotube array with a uniform pitch of 66 nm. Red area indicates the existence of strong attractive dielectrophoretic force while the blue area is related with repulsive force. ( d ) The calculated average dielectrophoretic force at the half-pitch position between neighbouring nanotubes as a function of pitch values. Red line plots the fitting to a logarithmic decay function of y = Ae − x / t , where t is the exponential time constant. Full size image Electrical properties of assembled nanotube arrays The electrical properties of assembled ultrahigh-density semiconducting nanotube arrays are assessed via their integration into active transistors. 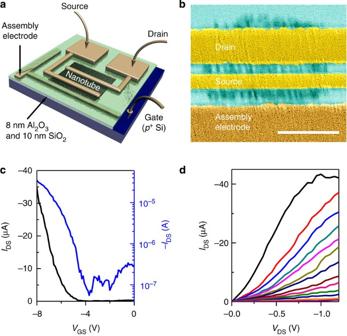Figure 4: FETs based on ultrahigh-density semiconducting nanotube arrays assembled using the fringing-field dielectrophoresis. (a,b) Schematic (a) and false-coloured SEM image (b) of a nanotube FET that incorporates purely semiconducting carbon nanotube arrays as channel. Device channel width is 1 μm and channel length is 100 nm. Scale bar, 500 nm. (c) Transfer characteristic of this transistor with drain–source current (IDS) plotted in both linear (left axis, black) and logarithmic (right axis, blue) scales. Gate–source bias (VGS) is swept between −8 and 0 V. Applied source–drain bias (VDS) is −0.5 V. (d) Current–voltage characteristic of this transistor with appliedVGSchanging from −8 to −2 V at a step of 0.25 V from top to bottom. Figure 4a schematically illustrates the device structure, with a SEM image shown in Fig. 4b . A 100-nm wide Ti/Pd/Au electrode, which is separated from the assembly electrode by 100 nm, serves as the source electrode. The device channel length is 100 nm. Since the average length of nanotubes used for assembly is around 600 nm, most nanotubes are able to directly bridge the source/drain electrodes. Al 2 O 3 (8 nm) deposited by atomic layer deposition plus 10 nm thermal silicon oxide are used as gate dielectrics with the heavily doped silicon substrate used as a back gate. The device channel width is 1 μm, defined by standard electron-beam (e-beam) lithography and oxygen plasma etching. Figure 4c plots the transfer characteristic of a device based on an array composed of purely semiconducting nanotubes, where the absence of even a single metallic nanotube is suggested by the high, c.a.~1,000, on/off current ratio. The current–voltage characteristics of the same device are depicted in Fig. 4d , showing an on-current density of 43 μA μm −1 and a peak transconductance ( g m ) of 52 μS μm −1 under a source–drain bias of −1 V and a gate overdrive voltage of −2 V. These results are a significant improvement over the previous best results of 10~15 μS μm −1 obtained under the same bias conditions from FETs built on assembled submonolayered semiconducting nanotube arrays [14] , [25] , despite a much thicker gate dielectric employed in current devices. Such performance advantage directly reflects the much improved material properties of nanotube arrays enabled by this fringing-field dielectrophoretic assembly technique. Our assembly process does not significantly affect the performance on per tube basis, with the average on-current per tube ~0.9 μA, close to the average on-current of ~1.3 μA measured for placed nanotubes [14] . It is likely still limited by the parasitic resistance at contacts, as evident from the strong super-linear behaviour at low bias shown in Fig. 4d , which indicates the existence of a significant barrier at the contacts. New strategies to improve the contact for densely packed nanotubes, such as converting from current side-bonded contacts to end-bonded structure using reactive contact metals, need to be established to further improve the performance of FETs constructed on ultrahigh-density nanotube arrays, where the contact area for each nanotube could be limited [36] . Figure 4: FETs based on ultrahigh-density semiconducting nanotube arrays assembled using the fringing-field dielectrophoresis. ( a , b ) Schematic ( a ) and false-coloured SEM image ( b ) of a nanotube FET that incorporates purely semiconducting carbon nanotube arrays as channel. Device channel width is 1 μm and channel length is 100 nm. Scale bar, 500 nm. ( c ) Transfer characteristic of this transistor with drain–source current ( I DS ) plotted in both linear (left axis, black) and logarithmic (right axis, blue) scales. Gate–source bias ( V GS ) is swept between −8 and 0 V. Applied source–drain bias ( V DS ) is −0.5 V. ( d ) Current–voltage characteristic of this transistor with applied V GS changing from −8 to −2 V at a step of 0.25 V from top to bottom. Full size image In summary, we have demonstrated the feasibility of assembling high-quality ultrahigh-density semiconducting nanotube arrays with very consistent pitch using the fringing-field dielectrophoresis. The field-focusing effect of fringing field leads to very strong electro-orientation torque to align nanotubes into well-ordered arrays with high degree of linearity. Moreover, the deposition of nanotubes is restricted within one submonolayer in a self-limited fashion as the fringing field above the substrate will be fully screened by the deposited nanotubes. Finally, following a similar mechanism, the inter-nanotube pitch is also self-limiting. These features allow us to achieve an ultrahigh density of ~50 nanotubes per μm, with a consistent pitch of 21±6 nm excluding significant formation of multilayer defects over a wide nanotube solution concentration window, as demonstrated in experiments and verified by numerical simulations. Transistors based on purely semiconducting nanotube arrays assembled by this method demonstrate high performance at both device and per tube level. We believe the high quality of assembled nanotube arrays, the easy implementation of the assembly process and the wide process window enabled by the unique self-limiting mechanism could make this fringing-field dielectrophoresis technique a robust nanomanufacturing method, and can be easily extended to pattern other nanomaterials or biomaterials. Preparation of nanotube aqueous solution Aqueous solution of single-walled carbon nanotubes was prepared by dispersing nanotube powders synthesized by arc-discharge method (Hanwha Nanotech, ASP-100F) in a 1% wt solution of SDS via horn sonication (20 min, 1 s pulse, 600 W, 99% amplitude, 20 kHz). The solution was further purified with a step-gradient centrifuge step utilizing 45% iodixanol (Sigma-Aldrich) solution with 0.25% SDS as a stopping layer at 287,700 g for 15 h using a Beckman Coulter Optima L-100 XP ultracentrifuge with a swinging bucket type rotor, to remove graphitic impurities and large bundles. The enrichment of semiconducting nanotubes was performed by passing the purified nanotube solution through a chromatographic column loaded with Sephacryl-200 (ref. 28 ). The solution divides into two distinct bands while passing through the column. The first band is blue-green in colour and rich in metallic nanotubes while the latter is red in colour and is primarily semiconducting. The 99% purity of semiconducting nanotube was confirmed with both absorption spectroscopy and direct electrical characterizations. Excessive surfactant in the solution was then removed via dialysis, where the nanotube solution was injected into a dialysis cartridge (Thermal Scientific, 10,000 molecular weight cut off) and soaked in a 1-L bucket of deionized water, which was replaced daily for 4 days. A final centrifuge step at 17,000 g was performed before use to remove large impurity particles. The concentration of nanotube solution was determined by the thermal gravimetric analysis. Device fabrication After assembling the semiconducting nanotube arrays, a standard e-beam lithography step was performed to pattern hydrogen silsesquioxane/poly(methyl methacrylate) bilayer resist into etch masks covering the active area of each device, which defined the device channel width, as all nanotubes outside of this area were removed by a subsequent oxygen plasma etching. After removing photoresist by hot acetone soaking, device source/drain electrodes were defined by another lithography step followed by lift-off of e-beam-evaporated Ti (0.2 nm)/Pd (15 nm)/Au (15 nm). Instrumentation Optical absorption spectrum of sorted nanotube solution was recorded with a Perkin Elmer Lambda 950 UV/Vis spectrometer. Thermal gravimetric analysis was performed using a Thermal Advantage Q50 equipment at a rate of 10 °C min −1 . Alternating voltage signal for assembly was applied using a Wavetek 188 function generator. SEM and AFM images were acquired with a Zeiss/LEO 1560 microscope and a Dimension 3000 instrument, respectively. Polarized Raman spectra were measured under an excitation wavelength of 532 nm, using the LabRAM ARAMIS micro-Raman setup. A Leica Vb6 e-beam writer was used to pattern photoresist. The electrical characterizations were carried out in a probe station using an Agilent B1500 parameter analyzer in air at room temperature. Simulations were performed using Comsol Multiphysics, a commercial partial differential equation solver that uses the finite-element method with adaptive meshing, error control and a variety of numerical solvers. How to cite this article: Cao, Q. et al . Fringing-field dielectrophoretic assembly of ultrahigh-density semiconducting nanotube arrays with a self-limited pitch. Nat. Commun. 5:5071 doi: 10.1038/ncomms6071 (2014).